Desktop nanofabrication with massively multiplexed beam pen lithography The development of a lithographic method that can rapidly define nanoscale features across centimetre-scale surfaces has been a long-standing goal for the nanotechnology community. If such a ‘desktop nanofab’ could be implemented in a low-cost format, it would bring the possibility of point-of-use nanofabrication for rapidly prototyping diverse functional structures. Here we report the development of a new tool that is capable of writing arbitrary patterns composed of diffraction-unlimited features over square centimetre areas that are in registry with existing patterns and nanostructures. Importantly, this instrument is based on components that are inexpensive compared with the combination of state-of-the-art nanofabrication tools that approach its capabilities. This tool can be used to prototype functional electronic devices in a mask-free fashion in addition to providing a unique platform for performing high-throughput nano- to macroscale photochemistry with relevance to biology and medicine. The pace of development in many areas of nanotechnology, physics, electronics, chemistry and biology is determined by the availability of reliable pattern generation tools. Therefore, a long-standing goal in these communities is the realization of a desktop nanofabrication tool that combines low-cost and high-resolution patterning with high-throughput operation. Such a tool would revolutionize the field in a manner analogous to the way that the desktop printer has revolutionized information transfer. However, desktop nanofabrication remains a formidable challenge because direct write systems available today, such as those that employ electron beam lithography (EBL) [1] , near-field optical lithography [2] , [3] , [4] , [5] , [6] , [7] , zone plate array lithography [8] , dip-pen nanolithography [9] , [10] and related molecular printing techniques [11] , [12] , [13] , [14] , impose tradeoffs between throughput, cost and feature size. The low cost and parallel nature of photolithography make it a promising candidate for desktop nanofabrication, but for this to be realized, diffraction-unlimited features must be attainable. There are many methods to circumvent the diffraction limit, including operating in the near-field regime [15] , utilizing two-photon processes [16] , incorporating plasmonic materials to locally enhance light [17] , [18] and constructing superlenses from negative index of refraction materials [19] . One promising technique that utilizes near-field apertures to overcome the diffraction limit is beam pen lithography (BPL) [6] , in which apertures with sub-wavelength dimensions at the tip of each gold-coated elastomeric pen in a massive array are used to perform scanning near-field optical lithography. However, there are two major challenges that have prevented BPL from being transitioned into a legitimate desktop nanofabrication tool: (1) all pens in the array act in unison, making this technique useful only for generating replicas of patterns, and (2) apertures are either constructed serially using a focused ion beam or in parallel using a mechanical stripping technique that yields >500 nm pores. Here, we report advances that address both of these issues and transform BPL into a real desktop tool capable of nanofabrication. This approach was made possible by combining BPL with a digital micromirror device such as those used in maskless lithography [20] , [21] and developing a novel strategy for coordinating the light addressing each pen with the motion of the pen array ( Fig. 1 and Supplementary Fig. S1 ). Once the light reaches the pen array, three structural aspects of the array [6] , [22] enable it to effectively perform near-field lithography: (1) a rigid and transparent glass backing layer allows light to reach the pens while structurally supporting the pen array, (2) the mechanical compliance of the polydimethylsiloxane pens allows them to be in gentle simultaneous contact with the surface and (3) the opaque gold coating and nanoscale size of the apertures in the array allow for nanoscale confinement of light. Using the resulting tool, we have fabricated centimetre-scale arrangements of nanoscale features to illustrate the ability of this actuated BPL approach to function as a general desktop nanofab. This transformative combination preserves the high spatial resolution of near-field optical lithography while gaining the ability to independently control the patterns generated by each pen in a massive and parallel fashion, creating a unified tool for constructing and studying nanomaterials. 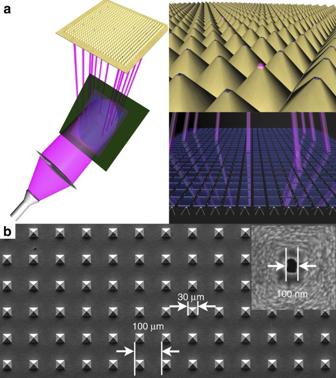Figure 1: Schematic of actuated BPL. (a) Schematic of the principle of operation of actuated BPL. A digital micromirror device (DMD) is illuminated with ultraviolet light, which is selectively directed onto the back of a near-field aperture array. (b) Scanning electron microscope (SEM) image of section of the BPL tip array. Each pyramidal pen in the array has a sub-wavelength aperture that has been opened in a parallel fashion. Figure 1: Schematic of actuated BPL. ( a ) Schematic of the principle of operation of actuated BPL. A digital micromirror device (DMD) is illuminated with ultraviolet light, which is selectively directed onto the back of a near-field aperture array. ( b ) Scanning electron microscope (SEM) image of section of the BPL tip array. Each pyramidal pen in the array has a sub-wavelength aperture that has been opened in a parallel fashion. Full size image Diffraction-unlimited nanopatterning The sub-wavelength apertures at the tip of each probe of a BPL pen array are crucial to the operation of actuated BPL and must be fabricated in a parallel and uniform fashion to preserve the low cost and scalable nature of this process. In a typical experiment, polymer pen arrays are moulded from Si masters and coated with an opaque layer (see Methods). To fabricate small and uniform apertures at the tip of each probe, we utilized a variant of a method that combines dry and wet etching [23] ( Supplementary Fig. S2 ) to controllably fabricate apertures with diameters of 103±12 nm ( Fig. 1b ). This important advance in BPL pen array fabrication allows for massively parallel diffraction-unlimited writing. As with any lithography system, it is important to establish the fundamental constitutive units from which patterns can be generated. In a typical experiment, a BPL pen array was mounted in a scanning probe lithography system and leveled with respect to a photoresist-coated Si wafer using an optical leveling procedure. To expose a region of the resist, the pens were brought into contact with the surface, and the back side of the pen array was illuminated with ultraviolet light with wavelength λ =405 nm while the array was held still for a specified exposure time. The sub-λ apertures block propagating light, and create an intensity profile that decays exponentially with distance from the aperture [3] , [24] . To optimize the exposure time, a dose test was performed in which the pen array wrote a series of dots ( Fig. 2a ) with exposure times between 2 and 4 s. At an effective exposure dose of 2 s, the dot features had an average diameter of 122±12 nm, which is substantially smaller than λ/2, demonstrating diffraction-unlimited performance. At longer exposure times, larger features were written, demonstrating control over feature size with exposure dose ( Fig. 2b ) [15] . In contrast to writing dots with the pens held still, moving the pens at a constant velocity across the sample while in contact allows one to write lines. Au lines with widths of 380±19, 842±17, 1,170±20 and 1,530±20 nm were written by scanning the tip array at 4, 2, 1 and 0.5 μm s −1 , respectively. In these experiments, the structures written by the pens were visualized by scanning electron microscopy after they had been coated with 5 nm of Cr and 25 nm of Au in a standard lift-off process. Interestingly, the root-mean-square line edge roughness of these features was 30 nm, highlighting the ability of actuated BPL to write high-quality lines. 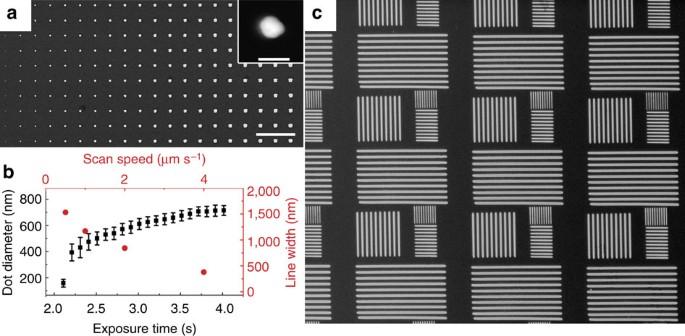Figure 2: Constitutive patterning units. (a) Dots written by a single pen in the BPL array. The exposure dose varies linearly from 2 s on the left to 4 s on the right, the inset shows the detailed morphology of a dot generated with a 2 s exposure. The scale bar is 5 μm and the scale bar in the inset is 100 nm. (b) Plots of feature diameter versus exposure dose (black square, bottom and left axes) and line width versus writing speed (red circle, top and right axes). Features with an average size of 122 nm were consistently written. Error bars represent the standard deviation in dot diameter, error in line width is smaller than the marker size. (c) Line patterns written at varying scan speed. The longest lines are 80 μm long. Figure 2: Constitutive patterning units. ( a ) Dots written by a single pen in the BPL array. The exposure dose varies linearly from 2 s on the left to 4 s on the right, the inset shows the detailed morphology of a dot generated with a 2 s exposure. The scale bar is 5 μm and the scale bar in the inset is 100 nm. ( b ) Plots of feature diameter versus exposure dose (black square, bottom and left axes) and line width versus writing speed (red circle, top and right axes). Features with an average size of 122 nm were consistently written. Error bars represent the standard deviation in dot diameter, error in line width is smaller than the marker size. ( c ) Line patterns written at varying scan speed. The longest lines are 80 μm long. Full size image Large-area arbitrary nanolithography Having established the core structures that actuated BPL can be used to write, we explored the potential of using its massively parallel and individually addressable nature to generate centimetre-scale arbitrary patterns composed of nanoscale features. The lithographic procedure entailed sequentially moving the pen array through an array of points on the sample while the digital micromirror device displayed images extracted from a master image. To achieve registry between the projected image and the pens, a novel alignment procedure ( Supplementary Fig. S3 ) and custom software were used ( Supplementary Fig. S4 ). To evaluate whether this technique could be used to generate centimetre-scale patterns composed of nanoscale features, a 8,100 pen array was used to generate a mosaic map of the world ( Fig. 3a ) wherein each tile of the world image ( Fig. 3c ) was a bitmap depicting the structure of a unique molecule from the PubChem database (for the high-resolution master image, see Supplementary Fig. S5 ). Importantly, this pattern was chosen to highlight the multiscale nature of patterning as the macroscale pattern (the map of the world) is composed of microscale objects (chemical formulae), which are in turn entirely composed of nanoscale dot features. The final pattern consists of 1.3 million dot features arranged to define 900 molecular structures in a 9 × 9 mm 2 area. In order to differentiate between molecules in the ‘land’ and ‘ocean’ regions of the world map, the exposure dose used to define the points in the land regions was twice that of the points in the ocean regions. After gold deposition and resist lift-off, the pattern consisted of 144±11 nm average diameter dot features in the regions corresponding to ocean ( Fig. 3d ) and 750±22 nm average diameter dot features written in the regions corresponding to land ( Fig. 3c ), all with a 1 μm pitch, demonstrating high quality control of light over the macro- to nanoscale. It is important to note that both the large and small features were written in the same experiment through control of the fraction of the total time that each mirror was activated. This pattern contains features that are too small to be fabricated using conventional optical techniques; it would be necessary to use EBL to even attempt to write such a pattern. 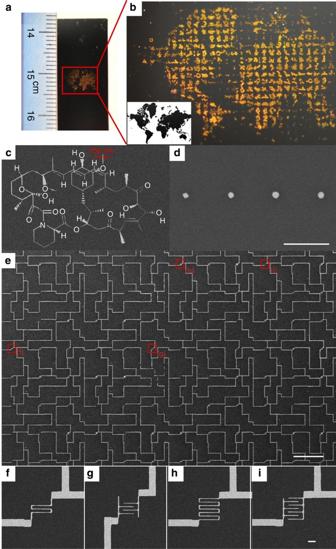Figure 3: Large-area arbitrary patterning with actuated BPL. (a) Photographic image of an arbitrary pattern 9 × 9 mm2in size, a portion of a ruler is shown for scale. (b) Magnified photograph of the pattern ina, with an inset depicting the image from which the mosaic was generated. (c) Scanning electron microscopy (SEM) image showing a molecule in the ‘land’ region. (d) SEM image showing a portion of a molecule in the ‘ocean’ region. The scale bar is 1 μm. (e) SEM image of an arbitrary pattern that consists of an array of planar resistors and capacitors with 120 nm line widths connected by an array of 2-μm-wide wires. This region of the pattern was written by contributions from 96 pens. The scale bar is 100 μm. (f–i) Four magnified examples of nanoscale circuit elements, whose positions are marked by red boxes in (e). The scale bar in (i) is 2 μm and the scale is the same for (f–i). Figure 3: Large-area arbitrary patterning with actuated BPL. ( a ) Photographic image of an arbitrary pattern 9 × 9 mm 2 in size, a portion of a ruler is shown for scale. ( b ) Magnified photograph of the pattern in a , with an inset depicting the image from which the mosaic was generated. ( c ) Scanning electron microscopy (SEM) image showing a molecule in the ‘land’ region. ( d ) SEM image showing a portion of a molecule in the ‘ocean’ region. The scale bar is 1 μm. ( e ) SEM image of an arbitrary pattern that consists of an array of planar resistors and capacitors with 120 nm line widths connected by an array of 2-μm-wide wires. This region of the pattern was written by contributions from 96 pens. The scale bar is 100 μm. ( f – i ) Four magnified examples of nanoscale circuit elements, whose positions are marked by red boxes in ( e ). The scale bar in ( i ) is 2 μm and the scale is the same for ( f–i ). Full size image As many example applications for which this tool would be useful require line features in addition to dot features, it is necessary to evaluate whether actuated BPL can be used to write large-area arbitrary patterns consisting of lines with sub-wavelength dimensions. To probe this, a patterning experiment was performed in which each probe was directed to write a 10 × 10 μm 2 resistor or capacitor at high resolution (50 nm pitch between points) and subsequently connect these elements together with a network of wires written in a 100 × 100 μm 2 region at low resolution (500 nm pitch between points). The result is a continuous network of ~2-μm-wide lines that span the entire surface ( Fig. 3e ) and connect an array of circuit elements comprised of 120±35-nm-wide wires ( Fig. 3f–i ). This pattern design was chosen as a proof-of-concept to mimic the architecture of small devices connected by larger interconnects commonly found in integrated circuits. Fabrication of functional devices The capabilities of actuated BPL were further evaluated by attempting to pattern functional circuits whose performance would be an indicator of successful patterning. To this end, arrays of Au serpentine resistors with varying lengths were fabricated on a Si wafer using actuated BPL ( Fig. 4a ). All resistors required the coordination of multiple pens with the largest requiring 15 pens and consisting of a 4-mm-long, 2-μm-wide continuous wire. Current–voltage characterization of 61 simultaneously patterned devices revealed that all measured devices exhibited Ohmic behaviour with resistances that depended linearly on the programmed line length ( Fig. 4b ). The sheet resistance of the resistors was computed by determining the slope of the linear fit and used to a sheet resistance of 0.32 Ω per square, in agreement with the tabulated value of 0.4 Ω per square for 50-nm-thick gold [25] . Furthermore, planar capacitors, inductors and surface acoustic wave (SAW) transducers were also patterned ( Fig. 4c ). It required 57 pens to write each capacitor, 51 pens to write each inductor and 110 pens to generate a pair of SAW transducers. To verify the function of the SAW transducers, they were combined with radio frequency amplifiers ( Supplementary Fig. S6 ) to form a delay line oscillator [26] , [27] whose resonance frequency of 11.9 MHz matches very well with the theoretical prediction of 12.3 MHz ( Fig. 4d ). 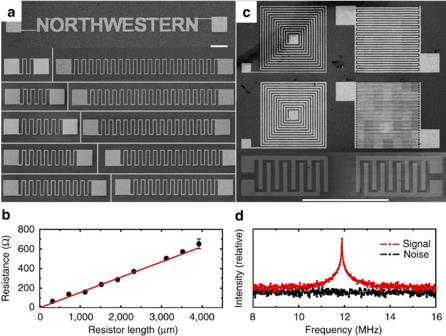Figure 4: Patterning active circuits with actuated BPL. (a) Serpentine resistors patterned by actuated BPL. Each resistor is formed of between 3 and 15 pens with the longest consisting of a 4 mm continuous line. The scale bar is 100 μm. (b) Plot of the resistance versus resistor length (black dots) with linear fitting (red line). Error bars represent the standard deviation in resistance from between 3 and 9 samples per resistor length. (c) Inductors, capacitors and a SAW sensor created by actuated BPL. The scale bar is 1 mm. (d) Frequency spectrum of the patterned SAW device. Noise spectrum was measured before the device was connected to the oscilloscope. Figure 4: Patterning active circuits with actuated BPL. ( a ) Serpentine resistors patterned by actuated BPL. Each resistor is formed of between 3 and 15 pens with the longest consisting of a 4 mm continuous line. The scale bar is 100 μm. ( b ) Plot of the resistance versus resistor length (black dots) with linear fitting (red line). Error bars represent the standard deviation in resistance from between 3 and 9 samples per resistor length. ( c ) Inductors, capacitors and a SAW sensor created by actuated BPL. The scale bar is 1 mm. ( d ) Frequency spectrum of the patterned SAW device. Noise spectrum was measured before the device was connected to the oscilloscope. Full size image Patterning in registry with existing nanostructures While piezoelectric control over the sample position allows features to be written with exceptionally high control over their position relative to one other, for many applications it is also necessary to generate patterns that are aligned to existing structures on a surface. To evaluate the potential of actuated BPL to pattern in registry with existing patterns, 150-nm-diameter semiconductor nanowires were dispersed on a silicon wafer with electrical contact pads and fiducial marks, imaged by optical microscopy ( Supplementary Fig. S7 ), and spin-coated with photoresist. Actuated BPL was then used to make electrical connection to the randomly dispersed nanowires by patterning electrical leads designed for this arrangement of nanowires ( Supplementary Fig. S8 ) after aligning the BPL pen array to the alignment marks on the sample, and writing the pattern ( Fig. 5a ). In this experiment, an array consisting of 729 (27 × 27) pens was used to write connections to 60 wires that had been located by optical microscopy. Patterning of this type, traditionally done by EBL [1] , shows how actuated BPL can be used to rapidly pattern in a mask-free fashion with registry to existing nanostructures. The success of this task was evaluated by measuring the number of patterned connections (59/60) and working devices after the lift-off process (40/60) ( Fig. 5b ). Finally, the electrical transport of the nanowire structures exhibited clear semiconducting behaviour ( Fig. 5c ), as one would expect for a working device. 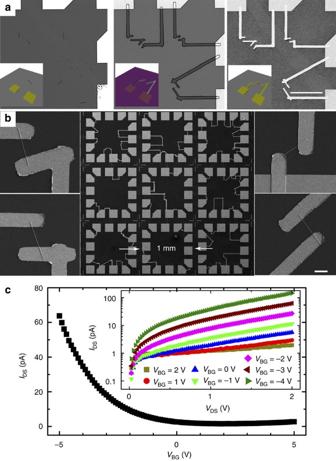Figure 5: Patterns written in registry with existing patterns and nanostructures. (a) The three-step process used to electrically connect randomly dispersed nanowires to existing electrodes: left, Si nanowires are distributed on a substrate with alignment marks and connection pads; middle, pattern was designed and transferred to the substrate by actuated BPL; right, 5 nm Cr and 150 nm Au were evaporated on the substrate and followed by lift-off. The scale bar is 100 μm. (b) Scanning electron microscopy image showing the whole substrate with the nanowires connected to the electrodes; the four insets show individual nanowire connections. The scale bar for the magnified panels is 5 μm. (c) Electrical characterization of a connected nanowire. Plot of the drain-source current (IDS) versus back gate voltage (VBG) with drain-source voltage of 1 V. The inset shows I–V curves of the device with different gate voltage, showing a characteristic transistor behaviour. Figure 5: Patterns written in registry with existing patterns and nanostructures. ( a ) The three-step process used to electrically connect randomly dispersed nanowires to existing electrodes: left, Si nanowires are distributed on a substrate with alignment marks and connection pads; middle, pattern was designed and transferred to the substrate by actuated BPL; right, 5 nm Cr and 150 nm Au were evaporated on the substrate and followed by lift-off. The scale bar is 100 μm. ( b ) Scanning electron microscopy image showing the whole substrate with the nanowires connected to the electrodes; the four insets show individual nanowire connections. The scale bar for the magnified panels is 5 μm. ( c ) Electrical characterization of a connected nanowire. Plot of the drain-source current ( I DS ) versus back gate voltage ( V BG ) with drain-source voltage of 1 V. The inset shows I–V curves of the device with different gate voltage, showing a characteristic transistor behaviour. Full size image Taken together, these data provide evidence for the first true desktop nanofabrication tool based upon easily fabricated BPL pen arrays, a novel strategy of actuation and a relatively simple scanning probe platform. This is the first such tool to allow one to rapidly generate structures of interest that span the macro-, micro- and nanoscales all in one experiment. The unique cantilever-free architecture makes this possible as light can be independently guided down the microscopic pyramid backing of each pen and confined through the nanoscale apertures in a high-throughout and high-yield fashion. Here, we show that features with sizes spanning 120 nm to several micrometres can be easily generated in a mask-free and scalable fashion; however, it is important to emphasize that these results represent only a proof-of-concept demonstration and not the fundamental limitation of the technique. For example, smaller apertures should enable sub-100 nm features [5] and improved engineering could enable writing speeds up to 2 mm 2 s −1 ( Supplementary Methods ). It is also worth noting that in addition to rapid prototyping applications in industrial or academic settings, this technique will also enable controlled light-mediated synthesis in localized spaces, which is becoming increasingly important in chemistry and biology. Pen array fabrication BPL pen arrays were fabricated starting with PPL pen arrays whose fabrication is described elsewhere [6] , [11] . The pen arrays were coated with 5 nm of Ti followed by 200 nm of Au to make them opaque, and then spin-coated with poly(methyl methacrylate) (PMMA 950 c7, MicroChem Inc., USA). Following coverage of the array, reactive ion etching was employed to isotropically etch the PMMA until the apexes of the pens were exposed. Subsequently, the gold at the apex of each pen was removed through a selective chemical etch (Gold Etchant TFA, Transense Company Inc., USA), leaving an aperture at the tip of each pen in the array. Residual PMMA was removed by rinsing in acetone. Lithographic procedure Si wafers with 500 nm of thermal oxide were spin-coated with lift-off resist (LOR Series, MicroChem Inc.) followed by S1805 (MicroChem Inc.) or AZ 1505 photoresist (MicroChemicals GmbH, Germany). Samples were then mounted in the actuated BPL apparatus and leveled following an optical leveling procedure. Patterns were then exposed in a frame-by-frame manner and subsequently developed in MF24A (MicroChem Inc.). Typically, 5 nm Cr and 15 nm Au were evaporated onto the sample followed by an overnight lift-off in Remover PG (MicroChem Inc.). Final patterns were characterized using atomic force microscopy (Dimension Icon, Bruker, USA), optical microscopy (Axiovert, Zeiss, USA) and scanning electron microscopy (S-4800-II and SU8030, Hitachi, Japan). Additional details The Supplementary Methods contains further details regarding the actuated BPL apparatus, the fabrication of BPL pen arrays, the alignment procedure used to align the projected light to the BPL pen arrays, the software control of actuated BPL and the general lithography procedure used to generate patterns. In addition, further details are provided regarding the design and testing of the SAW delay line oscillator and the nanowire connection procedure. How to cite this article: Liao, X. et al . Desktop nanofabrication with massively multiplexed beam pen lithography. Nat. Commun. 4:2103 doi: 10.1038/ncomms3103 (2013).